Quantum critical behaviour in confined SrTiO3quantum wells embedded in antiferromagnetic SmTiO3 Quantum phase transitions are driven by quantum fluctuations that alter the nature of the electronic quasiparticles, resulting in phenomena such as non-Fermi liquid behaviour. Oxide heterostructures offer fundamentally new ways of manipulating quantum criticality. Here, we report on non-Fermi liquid behaviour in thin SrTiO 3 quantum wells that are embedded in insulating, antiferromagnetic SmTiO 3 , as a function of temperature, quantum well thickness and SmTiO 3 layer thickness in superlattices. Such quantum wells contain very high sheet carrier densities on the order of one electron per pseudocubic planar unit cell. We show that the quantum well thickness is a tuning parameter for non-Fermi liquid behaviour. Increasing the thickness by a single atomic layer and coupling in superlattices recover the Fermi liquid behaviour. The critical exponents, the symmetry of the order parameter, the role of carrier densities and symmetry-lowering distortions are discussed, and the results are compared with those of quantum wells embedded in ferrimagnetic GdTiO 3 . Two-dimensional systems that are in the vicinity of a quantum critical point (QCP) have generated significant interest in condensed matter physics because they can promote the emergence of new ordered states, such as high-temperature superconductivity [1] , [2] . Interactions with critical fluctuations fundamentally alter the nature of electronic quasiparticles, causing phenomena such as non-Fermi liquid behaviour [3] , [4] , [5] . In bulk materials, quantum criticality is probed using magnetic fields, composition or pressure. Oxide heterostructures offer new opportunities to test the theoretical understanding of quantum criticality not possible with bulk materials. For example, critical fluctuations can be introduced controllably into an itinerant electron (or hole) system. Heterostructures also offer the exciting possibility of tuning symmetry through proximity effects [6] and dimensionality through electrostatic confinement and layer thicknesses. Moreover, systems can be doped electrostatically, which reduces the effects from disorder scattering, which can complicate the underlying physics [7] , [8] , [9] . Here we test these ideas using a model system of narrow SrTiO 3 quantum wells that are epitaxially embedded in an antiferromagnetic Mott insulator. These quantum wells contain electron densities that are sufficiently large for signatures of strong electron correlations to appear in transport [10] . Carriers are introduced electrostatically at Re TiO 3 /SrTiO 3 interfaces ( Re is a trivalent rare earth ion) [11] . At sufficiently small quantum well thicknesses, the Re TiO 3 insulator that interfaces the quantum well controls the symmetry of the quantum well and the (incipient) magnetism of the system, which are intimately linked [12] , [13] , [14] , [15] . Here we bring the electron system in proximity to a QCP by interfacing it with SmTiO 3 , which is an antiferromagnetic Mott insulator with a Neel temperature of ~50 K (ref. 16 ). We show that the critical behaviour can be manipulated by the quantum well thickness and by the spacing between the quantum wells in superlattices. The results show that these heterostructures provide a new and finely tunable platform to study emergent behaviour. Sample structures Two types of SmTiO 3 /SrTiO 3 /SmTiO 3 structures grown on (001) (LaAlO 3 ) 0.3 (Sr 2 AlTaO 6 ) 0.7 (LSAT) were investigated. The first contained single SrTiO 3 quantum wells embedded in 20-nm-thick insulating SmTiO 3 (10 nm on each side). In the following, the thickness of the SrTiO 3 quantum wells is specified by the number of SrO layers they contain, which ranged between 1- and 5-SrO layer(s) in this study. A second set of samples consisted of superlattices containing a single SrO layer in each repeat unit, denoted [ x SmTiO 3 /1-SrO] y , where x is the number of pseudocubic SmTiO 3 unit cells (u.c.) and y is the number of repeats. The pseudocubic lattice parameter of SmTiO 3 is ~0.39 nm (ref. 17 ). The SmTiO 3 thickness ( x ) was varied between 1.5 and 16 u.c in the superlattice samples. SmTiO 3 layers grown on LSAT substrates were insulating ( Supplementary Fig. 1 ). The resistivity of a 10-nm-thick SmTiO 3 film is ~0.08 Ω cm at 300 K and ~410 Ω cm at 100 K (they were too insulating to measure below 100 K), and thus presents a negligible contribution to the total sheet resistance of the single-quantum well structures. All quantum wells, even a single SrO layer, contained ~7 × 10 14 cm −2 mobile carriers, as a consequence of the charge mismatch at the interface (see ref. 11 and Supplementary Fig. 2 ). 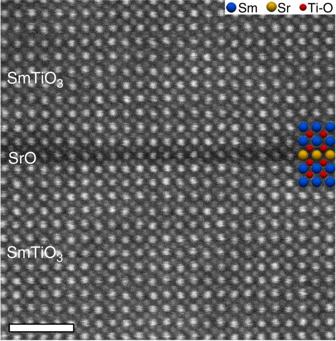Figure 1: Cross-section high-angle annular dark-field STEM image of a single SrO layer in SmTiO3. The SrO layer appears darker because of the lower atomic number of Sr relative to Sm. The image was corrected for sample drift. Scale bar, 2 nm. Figure 1 shows a representative atomic resolution scanning transmission electron microscopy (STEM) image of the single SrO layer. We have previously quantified interfacial roughness and structural distortions in these quantum wells as a function of quantum well thickness [14] . Quantum wells with thicknesses <3-SrO layers exhibited symmetry-lowering, orthorhombic-like structural distortions, although bulk SrTiO 3 is cubic at room temperature. Figure 1: Cross-section high-angle annular dark-field STEM image of a single SrO layer in SmTiO 3 . The SrO layer appears darker because of the lower atomic number of Sr relative to Sm. The image was corrected for sample drift. Scale bar, 2 nm. 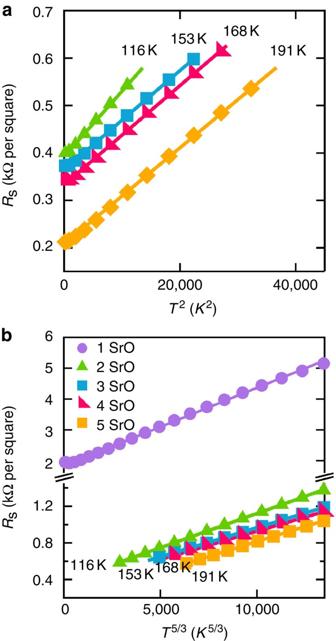Figure 2: Sheet resistances as a function of temperature for SrTiO3quantum wells of different thickness. (a)RSon aT2scale below the crossover temperature (see labels) to non-Fermi liquid behaviour. The lines are fits of formR0+AT2. (b)RSabove the crossover temperature (indicated) on aT5/3scale for quantum wells thicker than 1-SrO layer, and over the entireTrange for the 1-SrO quantum wells. The lines are fits of formR0+AT5/3. Only every fifth measured data point is shown for clarity. The thickness of the SrTiO3quantum wells is specified in terms of the number of SrO layers they contain. Full size image Phase diagram for single-quantum well structures Figure 2 shows the sheet resistance, R s , as a function of T n for the single-quantum well samples with different quantum well thicknesses, where T is the temperature. The exponent n was determined from fits to equations of form R s = R 0 + AT n , with R 0 , A and n as fit parameters (see Methods section). R 0 is the residual sheet resistance and A is the temperature coefficient. The lines in Fig. 2 are fits with n fixed to 2 and 5/3, respectively. The standard deviation (s.d.) for the free fits and the coefficients of determination ( R 2 values) for the fits with fixed n are extremely good (see Tables 1 and 2 ). Figure 2a shows that all quantum wells except the 1-SrO layer follow a T 2 (Fermi liquid) behaviour below a crossover temperature (given in the labels). Above the crossover temperature, the exponent in the temperature dependence changes to n ≈5/3 ( Fig. 2b ). R s of the 1-SrO layer follows a T 5/3 dependence with no crossover, as shown in Fig. 2b . All R s show an upturn at low temperatures that will be discussed below. Fits were only performed above the R s minimum. Non-Fermi liquid behaviour, that is, a temperature dependence of R s with an exponent n <2, is characteristic for an electron system that is near a QCP [5] . Figure 2: Sheet resistances as a function of temperature for SrTiO 3 quantum wells of different thickness. ( a ) R S on a T 2 scale below the crossover temperature (see labels) to non-Fermi liquid behaviour. The lines are fits of form R 0 + AT 2 . ( b ) R S above the crossover temperature (indicated) on a T 5/3 scale for quantum wells thicker than 1-SrO layer, and over the entire T range for the 1-SrO quantum wells. The lines are fits of form R 0 + AT 5/3 . Only every fifth measured data point is shown for clarity. The thickness of the SrTiO 3 quantum wells is specified in terms of the number of SrO layers they contain. Full size image Table 1 Fit results for single-quantum well structures with different thicknesses in different temperature ranges. Full size table Table 2 Fit results for superlattice structures with different SmTiO 3 spacer layer thicknesses in different temperature ranges. 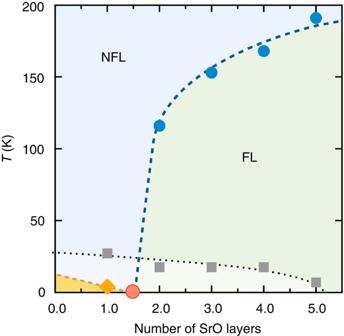Figure 3: Phase diagram showing Fermi- and non-Fermi liquid behaviour as a function of quantum well thickness. All samples contain a single-quantum well. The thickness is specified in terms of the number of SrO layers contained in the quantum well. The crossover temperatures (filled circles) are determined fromFig. 2and the fit results. Note that the 1-SrO quantum well shows no crossover within the temperature range analysed, so there is no data symbol for this sample. The diamond symbol indicates the temperature at which the positive magnetoresistance appeared for the 1-SrO layer sample. The approximate location of the QCP, if the transition to positive magnetoresistance is associated with a magnetically ordered phase, is indicated by the red dot. The squares indicate the temperature of the upturn inRS—no fits were performed below this temperature. All lines are a guide to the eye only and are not meant to indicate crossover temperatures for fractional layer thicknesses. FL, Fermi liquid; NFL, non-Fermi liquid. Full size table Figure 3 shows a phase diagram where the circles indicate the crossover temperatures between Fermi liquid and non-Fermi liquid regimes, determined from the fits, as a function of the number of SrO layers in the quantum wells. The 1-SrO quantum well shows non-Fermi liquid behaviour over a large temperature range, consistent with quantum fluctuations that persist to high temperatures. As can also be seen from Fig. 2 and Table 1 in the Methods section, the crossover temperature systematically decreases with decreasing quantum well thickness from ~190 K (5-SrO layers) to ~120 K (2-SrO layers) to no crossover above the temperature of the resistance upturn for the 1-SrO layer quantum well. Thus, the spatial dimension of the quantum well is the macroscopic tuning parameter for non-Fermi liquid behaviour. The phase diagram in Fig. 3 resembles the classic quantum critical ‘fan’, where, with increasing temperature, a larger region of the phase diagram is controlled by the QCP. Figure 3: Phase diagram showing Fermi- and non-Fermi liquid behaviour as a function of quantum well thickness. All samples contain a single-quantum well. The thickness is specified in terms of the number of SrO layers contained in the quantum well. The crossover temperatures (filled circles) are determined from Fig. 2 and the fit results. Note that the 1-SrO quantum well shows no crossover within the temperature range analysed, so there is no data symbol for this sample. The diamond symbol indicates the temperature at which the positive magnetoresistance appeared for the 1-SrO layer sample. The approximate location of the QCP, if the transition to positive magnetoresistance is associated with a magnetically ordered phase, is indicated by the red dot. The squares indicate the temperature of the upturn in R S —no fits were performed below this temperature. All lines are a guide to the eye only and are not meant to indicate crossover temperatures for fractional layer thicknesses. FL, Fermi liquid; NFL, non-Fermi liquid. Full size image Superlattices To further investigate the parameters that determine the non-Fermi liquid exponent, Fig. 4 shows results from superlattices, [ x SmTiO 3 /1-SrO] y that contain 1-SrO layer embedded in SmTiO 3 of varying thickness x . It is important to note at the outset that reducing the SmTiO 3 thicknesses results in a suppression of octahedral rotations in the SmTiO 3 (ref. 18 ). Since the octahedral tilts couple into the quantum well [14] , [19] , the quantum well structure and transport is correspondingly modified as well. Smaller tilts result in a larger bandwidth that also affects polaronic effects [16] . As can be seen from Fig. 4 , superlattices with thinner SmTiO 3 layers show systematically lower sheet resistances. Furthermore, magnetism, which is strongly coupled to the degree of octahedral tilts via the orbital polarization [17] , [20] , [21] , [22] , is gradually suppressed in thinner layers, as was previously shown for thin (<3.5 nm) ferrimagnetic GdTiO 3 layers [18] . As can be seen from Fig. 4 , all superlattices, except the one with 16 u.c. SmTiO 3 (~6.2 nm thickness), show Fermi liquid behaviour over a large temperature range. R s of the superlattice with 16 u.c. SmTiO 3 layers follows a T 4/3 dependence (high-quality fits to n of ~1.2 were also obtained, if the points near the resistance minimum were excluded). We will discuss the change in the critical exponent below. The combined studies suggest that disorder is not the origin of the non-Fermi liquid behaviour. For example, the same amount of disorder (that is, interface roughness or point defects) should be present in all samples, independent of the spacing between the quantum wells. Furthermore, n =2 for all quantum wells in GdTiO 3 (ref. 10 and Supplementary Table 1 ), which are grown under very similar conditions and show similar interface roughness [14] . 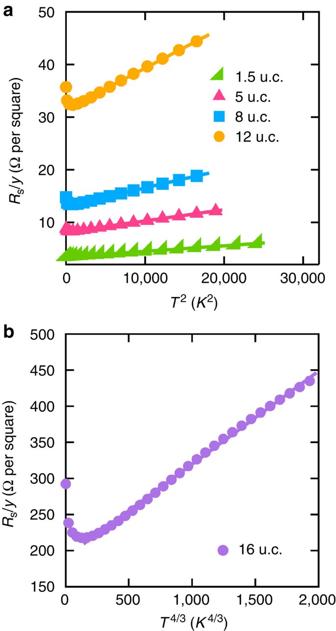Figure 4:RSas a function of temperature for the [xSmTiO3/1-SrO]ysuperlattices. RSis normalized by the number of quantum wells,y. The SmTiO3thickness (x) is given in legends in the number of pseudocubic u.c.’s. The number of repeats werey=14 forx=1.5, 5 and 8;y=8 forx=12; andy=6 for 16. A lowerywas chosen for thicker SmTiO3layers due to the onset of strain relaxation. (a) Data on aT2scale. The lines are fits of formR0+AT2. (b) Data for the superlattice with 16-u.c.-thick SmTiO3layers as a function ofT4/3. The line is a fit of formR0+AT4/3. Only every third measured data point is shown for clarity. Figure 4: R S as a function of temperature for the [ x SmTiO 3 /1-SrO] y superlattices. R S is normalized by the number of quantum wells, y . The SmTiO 3 thickness ( x ) is given in legends in the number of pseudocubic u.c.’s. The number of repeats were y =14 for x =1.5, 5 and 8; y =8 for x =12; and y =6 for 16. A lower y was chosen for thicker SmTiO 3 layers due to the onset of strain relaxation. ( a ) Data on a T 2 scale. The lines are fits of form R 0 + AT 2 . ( b ) Data for the superlattice with 16-u.c.-thick SmTiO 3 layers as a function of T 4/3 . The line is a fit of form R 0 + AT 4/3 . Only every third measured data point is shown for clarity. 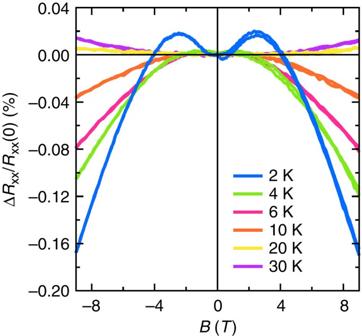Figure 5: Temperature dependence of the magnetoresistance of the single SrO layer quantum well. Bwas swept from +9T to −9T and back to +9T.Bwas in the plane of the film and the current was orthogonal toB. Full size image Low-temperature magnetoresistance Figure 5 shows the magnetoresistance of a 1-SrO single-quantum well sample. The magnetic field ( B ) was in the plane of the film and the current was orthogonal to B . Below ~20 K, the magnetoresistance changes sign from weakly positive to negative. The magnetoresistance changes again below ~4 K. At 2 K, the magnetoresistance is positive up to a critical field, B c (~2.5 T), then becomes negative for B > B c . As shown in Supplementary Fig. 3 , the positive ‘dip’ becomes very weak as the thickness of the quantum well is increased by just 1-SrO layer and vanishes for thicker quantum wells. Figure 5: Temperature dependence of the magnetoresistance of the single SrO layer quantum well. B was swept from +9T to −9T and back to +9T. B was in the plane of the film and the current was orthogonal to B . Full size image Several important questions arise, namely (i) the origin of the non-Fermi liquid exponents, n ≈5/3 in the single-quantum well samples and n ≈4/3 in the superlattices; (ii) the nature of any ordered phase in the system; and (iii) the mechanism(s) by which the quantum well thickness can act as a tuning parameter for quantum criticality. We first turn to the critical exponent. In the theory of quantum phase transitions, n is determined by the symmetry of the order parameter and by the dimensionality of the fluctuations [2] . A value of 5/3 observed for the quantum wells embedded in thick SmTiO 3 is predicted for a three-dimensional (3D) ferromagnet [23] . This appears to be inconsistent with a two-dimensional (2D) electron system [13] , [24] , [25] that is in proximity to an antiferromagnetic QCP. However, it is important to note that ‘ferromagnet’ in the theories refers to an order wavevector Q =(0,0,0). Thin quantum wells and SmTiO 3 both have orthorhombic-like symmetry, with a u.c. that is doubled along the parent cubic axes [14] . Thus, the order vector is not Q =(½,½,½) as for a simple cubic antiferromagnet, but Q =(0,0,0), when referred to the orthorhombic cell. Quantum well superlattices consisting of 1-SrO layers embedded in 16 u.c. SmTiO 3 layers exhibit an n of 4/3, which is the value expected for a 2D system with Q =(0,0) (ref. 23 ). Thus, it appears that confinement (or narrowing) of the SmTiO 3 layers reduces the dimensionality of the fluctuations, which determines n , somewhat independent from the dimensionality of the quasiparticles. Differences in the dimensionalities of quasiparticle and collective behaviour has also been observed in bulk materials [26] . However, further investigations are needed to confirm the interpretation of the change in the exponent in the superlattices, since the transport properties are clearly modified. For thinner SmTiO 3 layers in the superlattices, reduced octahedral tilts and/or more extensive coupling between the quantum wells drive the system further from the QCP, recovering Fermi liquid behaviour. We next turn to the question whether there is an itinerant magnetically ordered phase, as was found previously in narrow GdTiO 3 /SrTiO 3 /GdTiO 3 quantum wells [13] . For the 1-SrO quantum wells, positive magnetoresistance, that is, an increase of scattering with increase in B , appears below ~4 K. In antiferromagnets, positive magnetoresistance can arise from the moments aligned antiparallel to B [27] , and in spin density wave (SDW) systems it is because of the suppression of the SDW by the magnetic field that enhances the spin scattering. Positive magnetoresistance has been observed in many SDW systems [28] , [29] , [30] . This points to the QCP being located approximately between the 1- and 2-SrO layer quantum wells, as indicated in Fig. 3 . Further investigations are, however, clearly needed to investigate the presence and type of magnetic order in the 1-SrO layers. All samples show an upturn in the resistance and negative magnetoresistance ( Fig. 5 and Supplementary Fig. 3 ) at low T , which was also seen in quantum wells in GdTiO 3 (ref. 13 ). The temperature of the upturn is indicated by the dotted line in Fig. 3 . Nearly quadratic, isotropic negative magnetoresistance is characteristic for scattering due to spin fluctuations, which results in an increase in the resistance. The fluctuations are suppressed by B , decreasing the resistance. Even for wider quantum wells, a significant portion of the high-density electron system is located close to the interface with the insulating magnet (see ref. 25 and references cited therein). We tentatively attribute the negative magnetoresistance to scattering from those moments. The correction to the resistance becomes less pronounced for thicker quantum wells owing to their lower resistance and a larger fraction of the electron gas being located further away from the interface. We thus conclude that it is a separate effect that adds some complexity, but does not affect the main conclusions. Weak localization can also produce a negative magnetoresistance in 2D systems [31] and has been observed in SrTiO 3 (refs 32 , 33 , 34 , 35 ), but it only appears as a correction to the resistances close to strong localization ( R S ~25 kΩ per square) and is highly anisotropic. Finally, we discuss how the quantum well thickness (number of SrO layers) can act as a tuning parameter for quantum criticality. Reducing the quantum well thickness has two important consequences, and it is likely that both are important: first, it increases the 3D carrier density, which is essential for bringing the quantum well into a regime where on-site Coulomb interactions become relevant [10] , [15] ; and second, it introduces octahedral tilts into the quantum well [14] , [19] . For example, reducing the thickness of the quantum well from 2-SrO layers to 1-SrO layer causes the number of TiO 2 layers, over which ~1 electron per pseudocubic planar u.c. is distributed, to change from three to two (this count includes the interfacial TiO 2 layers), which corresponds to a large change in the 3D carrier density in the quantum well. The change in 3D carrier density is furthermore accompanied by a change in the symmetry of the quantum well. In particular, STEM studies have shown that structural distortions can be detected in the quantum wells with 2-SrO layers [14] . The symmetry change can have important consequences for the charge per u.c. and the correlation physics of the quantum well [15] . A comparison with results from GdTiO 3 /SrTiO 3 /GdTiO 3 quantum wells, which contain the same carrier density, is instructive. There, we also observe a similar thickness sensitivity in the phase diagram, namely, a change by just 1-SrO layer (from 3- to 2-SrO layers) that resulted in an abrupt metal–insulator transition to a self-trapped small polaron gas, accompanied by several orders of magnitude resistance change, and an abrupt transition to a lower-symmetry phase [10] , [14] , [19] , [36] . Quantum wells in GdTiO 3 with thicknesses just above the metal-to-insulator transition are ferromagnetic and mass enhancement is seen in transport, but they do not deviate from Fermi liquid behaviour (refs 10 , 13 ; Supplementary Fig. 4 and Supplementary Table 1 ). The ferromagnetism in the quantum wells is clearly distinct from the magnetism in the GdTiO 3 (ref. 13 ), that is, representing its own magnetic phase. In contrast, the SmTiO 3 /SrTiO 3 /SmTiO 3 quantum wells show no mass enhancement ( Supplementary Fig. 5 ), significantly smaller distortions in the quantum well [14] , no metal–insulator transition and quantum criticality. In general, there is a strong coupling between orbital order (or polarization), which correlates with the type of magnetic order [17] , [37] , [38] , [39] , and the degree of structural distortions in these materials. Thus, it is likely that the degree of lattice distortion, which is determined by the adjacent Re TiO 3 for sufficiently thin quantum wells and is tuned by changing the quantum well thickness or the thickness of the SmTiO 3 spacer layers in the superlattices, determines the orbital polarization and thereby the nature of and the proximity to the magnetically ordered state in the phase diagram. Interestingly, only proximity to an itinerant antiferromagnetic—not ferromagnetic—phase results in non-Fermi liquid behaviour. Clearly, further theoretical and experimental studies are needed to better understand the effect of the microscopic parameters on interactions with low-energy excitations, and the nature and relative roles of magnetic and orbital order and fluctuations in both systems. In summary, we have shown that 2D, high-density electron systems in oxide heterostructures can be tuned into quantum criticality by changing the dimensionality of the itinerant carrier system in the quantum well, which influences both the 3D carrier density and the symmetry of the quantum well, resulting in a classical quantum critical fan diagram. Analysis of the critical exponents indicated that the heterostructure parameters, in particular the spacing between the quantum wells, can be used to control the dimensionality of the critical fluctuations. The heterostructures investigated here allow for exploration of the physics of non-Fermi liquid behaviour, for example, by introducing more complex spin states and fluctuations. In analogy with bulk materials, other QCPs may exist nearby, and may be accessible with other tuning parameters available in heterostructures, such as strain, interface orientation or a change in carrier density. Sample preparation and electrical measurements SmTiO 3 /SrTiO 3 /SmTiO 3 structures were grown by hybrid molecular beam epitaxy [11] on (001) LSAT substrates. The superlattices were capped with SmTiO 3 . The quantum well thickness was confirmed using transmission electron microscopy. Contacts were deposited by electron beam evaporation using shadow masks for electrical measurements in either Van der Pauw (as-grown 1 × 1 cm 2 samples) or Hall bar geometry, and consisted of 40 nm Ti/400-nm Au, with the Au being the top layer. Resistance data were collected using a Physical Property Measurement System (Quantum Design PPMS Dynacool). Samples measured in Hall bar geometry were also measured in Van der Pauw geometry before processing them into Hall bar structures, and the two measurements agreed quantitatively. The data shown in Figs 2 and 5 is from two different 1-SrO quantum well structures, which showed similar transport properties and critical exponents n . Data fitting All fits of the temperature-dependent resistance were performed using a Levenberg–Marquardt non-linear least squares method (IGOR Pro data analysis software). The Tables 1 and 2 summarize the results obtained from fits of the temperature dependence of the R S for the SmTiO 3 /SrTiO 3 /SmTiO 3 single-quantum wells ( Table 1 ) and [ x SmTiO 3 /1-SrO] y superlattices ( Table 2 ). The s.d. for each fit parameter are shown. Also shown are the R 2 values for the lines shown in Figs 2 and 4 in the main text, which are linear fits using the n values stated in the Tables. How to cite this article: Jackson, C. A. et al. Quantum critical behaviour in confined SrTiO 3 quantum wells embedded in antiferromagnetic SmTiO 3 . Nat. Commun. 5:4258 doi: 10.1038/ncomms5258 (2014).